A mouse model for a partially inactive obesity-associated humanMC3Rvariant We previously reported children homozygous for two MC3R sequence variants (C17A+G241A) have greater fat mass than controls. Here we show, using homozygous knock-in mouse models in which we replace murine Mc3r with wild-type human ( MC3R hWT/hWT ) and double-mutant (C17A+G241A) human ( MC3R hDM/hDM ) MC3R , that MC3R hDM/hDM have greater weight and fat mass, increased energy intake and feeding efficiency, but reduced length and fat-free mass compared with MC3R hWT/hWT . MC3R hDM/hDM mice do not have increased adipose tissue inflammatory cell infiltration or greater expression of inflammatory markers despite their greater fat mass. Serum adiponectin levels are increased in MC3R hDM/hDM mice and MC3R hDM/hDM human subjects. MC3R hDM/hDM bone- and adipose tissue-derived mesenchymal stem cells (MSCs) differentiate into adipocytes that accumulate more triglyceride than MC3R hWT/hWT MSCs. MC3R hDM/hDM impacts nutrient partitioning to generate increased adipose tissue that appears metabolically healthy. These data confirm the importance of MC3R signalling in human metabolism and suggest a previously-unrecognized role for the MC3R in adipose tissue development. The murine melanocortin 3 receptor ( Mc3r ) plays an important role in regulating energy homeostasis [1] . Homozygous Mc3r knockout mice have a phenotype distinct from those of ob/ob or Mc4r knockouts [2] because Mc3r knockout mice exhibit greater fat mass with reduced fat-free mass, so that total body weight is not notably increased. Mc3r knockout mice show greater feeding efficiency (the ratio of weight gain to energy intake); they are described as hypophagic or normophagic relative to controls and appear to maintain normal metabolic rate [1] . Recent studies have also reported impaired fasting-induced lipolysis and corticosterone secretion [3] as well as potential dysregulation of mesolimbic dopaminergic reward systems [4] in Mc3r knockout mice. Linkage studies indicate that the human MC3R locus is associated with body weight [5] . Coding sequence variants that may be associated with obesity have also been reported in human MC3R [6] , [7] , [8] , [9] , [10] . A heterozygous missense sequence variant Ile183Asn (I183N) that inactivates MC3R function [11] , [12] was identified in two individuals [7] . Other variants, including C17A (Thr6Lys) and G241A (Val81Ile) have not been found individually to affect signal transduction [12] or be associated with body weight [6] , [8] , [9] , [10] . We and others have reported that homozygosity for the C17A+G241A MC3R haplotype is associated with childhood obesity and higher fat mass than observed for wild type or heterozygous children [13] , [14] , [15] , although this result has not been replicated among adults [16] and some in vitro data suggest that the major start site for translation for MC3R may begin at a second in-frame ATG that is downstream of C17A, placing C17A in the 5′ untranslated region [17] , [18] . However, some in vitro studies have found translation is possible from the first ATG [19] and have suggested that the C17A+G241A hMC3R may be partially inactive, with significantly fewer surface receptor binding sites, decreased signal transduction and less protein expression [13] , [15] . It remains unclear whether C17A+G241A MC3R affects energy homeostasis, given the genetic heterogeneity of humans in the extant studies. To characterize the potential effects of these gene variants on body weight, energy balance and metabolism, we therefore generated and compared two novel homozygous knock-in mouse models, replacing the murine Mc3r with either wild-type human MC3R ( MC3R hWT/hWT ) or the double-mutant C17A+G241A human MC3R ( MC3R hDM/hDM ), finding greater adiposity but without marked metabolic derangements in MC3R hDM/hDM . Validation of replacement of Mc3r in knock-in mice The strategy and targeting vector used to replace murine Mc3r with human MC3R are shown in Supplementary Fig. 1 . Direct sequencing after PCR amplification of genomic DNA of homozygous mice confirmed that murine Mc3r genes were replaced with human wild-type or double-mutant (C17A+G241A) MC3R and that there were no other genomic sequence differences introduced in the 6.17-kB targeted region. Only human MC3R messenger RNA (mRNA) expression in the hypothalamus was found for homozygous knock-in mice by quantitative RT–PCR performed using mouse- and human-specific primers ( Fig. 1a–d ). Western analysis confirmed MC3R was expressed in total hypothalamic protein lysates from both homozygous knock-in models ( Fig. 1e,f ). 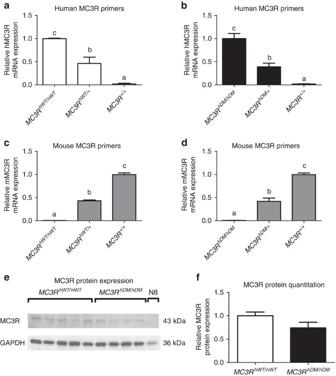Figure 1: Validation of mouseMC3Rreplacement by humanMC3R. Quantitative real-time PCR for relative hypothalamic mRNA expression normalized by β-actin expression by the 2–ΔΔCt method (n=3/group) in 4-month-old female C57BL/6 mice (MC3R+/+) or knock-in mice that were homozygous (MC3RhWT/hWT) or heterozygous (MC3RhWT/+) for the common alleles for the humanMC3Ror homozygous (MC3RhDM/hDM) or heterozygous (MC3RhDM/+) for the humanMC3Rsequence variants C17A+G241A. Expression was determined using human-specificMC3Rprimers (a,b) and mouse-specificMC3Rprimers (c,d).MC3Rprotein expression (e) was measured by western blotting (forMC3RhWT/hWTn=5; forMC3RhDM/hDMn=4) in homozygous mice and in the hypothalamic N8 murine cell line, which does not express MC3R mRNA. MC3R protein expression adjusted for GAPDH was quantified using Image J (f). Data are represented as mean±s.e.m. A different letter represents significant differences atP<0.05 compared with the other groups. Similar results were found for male mice (data not shown). Groups were compared by one-way analysis of variance followed by Bonferroni post-tests (a–d) and Student'st-test (two-tailed) (f). Figure 1: Validation of mouse MC3R replacement by human MC3R . Quantitative real-time PCR for relative hypothalamic mRNA expression normalized by β-actin expression by the 2–ΔΔCt method ( n =3/group) in 4-month-old female C57BL/6 mice ( MC3R +/+ ) or knock-in mice that were homozygous ( MC3R hWT/hWT ) or heterozygous ( MC3R hWT/+ ) for the common alleles for the human MC3R or homozygous ( MC3R hDM/hDM ) or heterozygous ( MC3R hDM/+ ) for the human MC3R sequence variants C17A+G241A. Expression was determined using human-specific MC3R primers ( a , b ) and mouse-specific MC3R primers ( c , d ). MC3R protein expression ( e ) was measured by western blotting (for MC3R hWT/hWT n =5; for MC3R hDM/hDM n =4) in homozygous mice and in the hypothalamic N8 murine cell line, which does not express MC3R mRNA. MC3R protein expression adjusted for GAPDH was quantified using Image J ( f ). Data are represented as mean±s.e.m. A different letter represents significant differences at P <0.05 compared with the other groups. Similar results were found for male mice (data not shown). Groups were compared by one-way analysis of variance followed by Bonferroni post-tests ( a – d ) and Student's t -test (two-tailed) ( f ). Full size image Body composition To examine the effects of double-mutant human MC3R on body composition, we compared body weight and body composition of littermate female and male C57BL/6 mice without human gene insertion ( MC3R +/+ , n =16) with female and male knock-in mice that were heterozygous ( MC3R hWT/+ ) or homozygous ( MC3R hWT/hWT ) for the wild-type human MC3R and with female and male mice that were heterozygous ( MC3R hDM/+ ) or homozygous ( MC3R hDM/hDM ) for the double-mutant human MC3R . On chow diets, female and male MC3R hDM/hDM mice had significantly greater body weight compared with MC3R hWT/hWT or MC3R +/+ mice ( Supplementary Fig. 2 ). No differences in body weight were observed among MC3R +/+ , MC3R hWT/+ , MC3R hWT/hWT or MC3R hDM/+ mice ( Supplementary Fig. 2 ). On a 45% high-fat diet, female and male MC3R hDM/hDM mice also had significantly greater body weight compared with MC3R hWT/hWT mice ( Supplementary Fig. 3 ). Body composition was notably affected by MC3R hDM/hDM . On both chow and high-fat diets, both female ( Fig. 2a–e ) and male ( Supplementary Fig. 4a–e ) MC3R hDM/hDM mice had significantly greater body fat mass, but reduced fat-free mass, compared with MC3R hWT/hWT mice. The increased fat mass in high-fat-fed MC3R hDM/hDM appeared not to be fat-depot specific, as evidenced by increased epididymal fat, subcutaneous flank fat and interscapular brown fat depots ( Supplementary Fig. 5a–c ). Although haematoxylin and eosin (H&E) staining showed that lipid accumulation appeared to be increased in brown adipose tissue of MC3R hDM/hDM , UCP1 protein expression was maintained in MC3R hDM/hDM mice ( Supplementary Fig. 6a–d ). There was no significant difference in liver weight between high-fat-diet-treated mice ( Supplementary Fig. 5d ). H&E staining and liver triglyceride measurements after an overnight fast showed no significant differences in triglyceride accumulation between groups in the high-fat-fed condition ( Supplementary Fig. 7a–c ), suggesting that liver steatosis is not markedly exacerbated despite the greater fat mass of MC3R hDM/hDM mice. 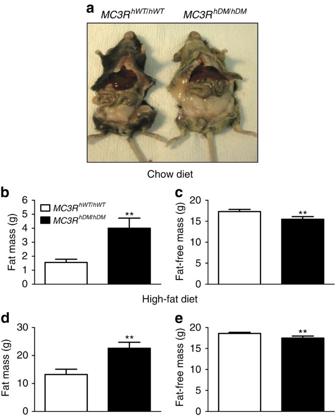Figure 2: Greater fat mass and reduced fat-free mass inMC3RhDM/hDMmice. (a) Female (5-month old)MC3RhDM/hDMmice had increased adiposity compared withMC3RhWT/hWT. (b,c) FemaleMC3RhWT/hWT(n=7, open bars) orMC3RhDM/hDM(n=10, closed bars) mice were fed chow diet or (d,e) high-fat diet (MC3RhWT/hWTn=6;MC3RhDM/hDMn=9) for 2 months. Body fat mass and fat-free mass were measured by MRI at age 2–3 months and 4–5 months for chow-fed and high-fat-fed mice, respectively. Data are represented as mean±s.e.m. *P<0.05 and **P<0.01MC3RhDM/hDMversusMC3RhWT/hWTmice. Groups were compared by Student'st-tests (two-tailed) (b–e). Figure 2: Greater fat mass and reduced fat-free mass in MC3R hDM/hDM mice. ( a ) Female (5-month old) MC3R hDM/hDM mice had increased adiposity compared with MC3R hWT/hWT . ( b , c ) Female MC3R hWT/hWT ( n =7, open bars) or MC3R hDM/hDM ( n =10, closed bars) mice were fed chow diet or ( d , e ) high-fat diet ( MC3R hWT/hWT n =6; MC3R hDM/hDM n =9) for 2 months. Body fat mass and fat-free mass were measured by MRI at age 2–3 months and 4–5 months for chow-fed and high-fat-fed mice, respectively. Data are represented as mean±s.e.m. * P <0.05 and ** P <0.01 MC3R hDM/hDM versus MC3R hWT/hWT mice. Groups were compared by Student's t -tests (two-tailed) ( b – e ). Full size image Crown-rump length of MC3R hDM/hDM mice was slightly, but significantly, shorter than that of MC3R hWT/hWT mice ( Supplementary Fig. 8a,b ). We used dual-energy X-ray absorptiometry (DXA) to further characterize body composition. Body fat mass was significantly increased without apparent differences in lean mass ( Supplementary Fig. 9a–c ), although percentage lean mass was significantly reduced in both female and male MC3R hDM/hDM mice ( Supplementary Fig. 9d ). By DXA, we found no differences in total mouse bone mineral density (BMD; Supplementary Fig. 9e ), although, in accord with their decreased length, total bone mineral content and bone area were significantly reduced in MC3R hDM/hDM mice ( Supplementary Fig. 9f,g ). No skeletal malformations were identified in MC3R hDM/hDM mice. To study bone microarchitecture more precisely, we performed micro computed tomography (CT) analysis using femurs from MC3R hWT/hWT and MC3R hDM/hDM mice. Femurs from MC3R hDM/hDM mice had reduced length ( Supplementary Fig. 8c–e ) as well as lower BMD in whole bone and trabecular bone without significant differences in cortical BMD ( Supplementary Fig. 8f ). Furthermore, MC3R hDM/hDM mice exhibited a trend towards lower trabecular number and significantly decreased trabecular bone-volume fraction, trabecular bone thickness, cortical area fraction and average cortical thickness, compared with MC3R hWT/hWT mice ( Fig. 3a–e,g,h ). Analysis of femurs ( Fig. 3f ) found the medullary cavity area in cortical regions was also significantly increased in MC3R hDM/hDM mice, suggesting there might be increased marrow fat. We therefore isolated bone marrow from femurs, finding significantly greater marrow triglycerides in MC3R hDM/hDM mice ( Supplementary Fig. 10 ). These data indicate reduced bone mass and increased bone marrow fat in MC3R hDM/hDM compared to MC3R hWT/hWT mice. Reduced bone size and increased marrow fat thus contribute to the decreased fat-free mass and increased fat mass of MC3R hDM/hDM mice. 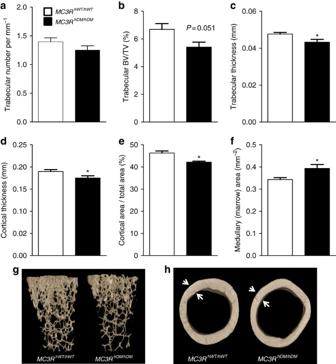Figure 3: Micro-CT shows decreased bone in femurs ofMC3RhDM/hDMmice. (a) Trabecular number (per mm) of chow-fed female (12-week old)MC3RhDM/hDMandMC3RhWT/hWTmice. (b) Trabecular bone-volume fraction: Trabecular Bone Volume/Total Volume (BV/TV), (c) Trabecular thickness, (d) average cortical thickness, and (e) Cortical area per Total area fraction were reduced inMC3RhDM/hDM; (f) Medullary (marrow) area was increased inMC3RhDM/hDM; (g) representative reconstructed 3D images of femur trabecular bones; (h) representative cross-sectional cortical bones (h). Data are represented as mean±s.e.m.;MC3RhWT/hWTn=7;MC3RhDM/hDMn=8. *P<0.05MC3RhDM/hDMversusMC3RhWT/hWTmice. Groups were compared by Student'st-tests (two-tailed) (a–f). Figure 3: Micro-CT shows decreased bone in femurs of MC3R hDM/hDM mice. ( a ) Trabecular number (per mm) of chow-fed female (12-week old) MC3R hDM/hDM and MC3R hWT/hWT mice. ( b ) Trabecular bone-volume fraction: Trabecular Bone Volume/Total Volume (BV/TV), ( c ) Trabecular thickness, ( d ) average cortical thickness, and ( e ) Cortical area per Total area fraction were reduced in MC3R hDM/hDM ; ( f ) Medullary (marrow) area was increased in MC3R hDM/hDM ; ( g ) representative reconstructed 3D images of femur trabecular bones; ( h ) representative cross-sectional cortical bones ( h ). Data are represented as mean±s.e.m. ; MC3R hWT/hWT n =7; MC3R hDM/hDM n =8. * P <0.05 MC3R hDM/hDM versus MC3R hWT/hWT mice. Groups were compared by Student's t -tests (two-tailed) ( a – f ). Full size image Energy intake, feeding efficiency and energy expenditure In both chow and high-fat diet-fed conditions, energy intake, assessed over 2 weeks and adjusted for fat-free mass, was significantly increased ( P =0.044 and 0.048 for chow and high-fat diet-fed conditions, respectively) in female MC3R hDM/hDM versus MC3R hWT/hWT mice ( Supplementary Table. 1a,b ). Similar results were found in chow-fed male MC3R hDM/hDM mice (data not shown). After adjusting for total body weight, energy intake was still significantly increased in high-fat-fed, but not chow-fed MC3R hDM/hDM mice ( Supplementary Table 1a,b ). In both chow and high-fat diet-fed conditions, food intake was not different between groups after adjusting separately for both fat and fat-free mass ( Supplementary Table 1a,b ). Because increased feeding efficiency has been observed in Mc3r knockout mice [1] , we examined feeding efficiency in both female and male MC3R hWT/hWT and MC3R hDM/hDM mice fed ad libitum . Feeding efficiency (weight gain relative to energy intake) was markedly higher in female MC3R hDM/hDM mice versus MC3R hWT/hWT in both chow and high-fat-fed conditions ( Fig. 4a,b ). Similar results were found in male MC3R hDM/hDM mice (data not shown). To examine feeding efficiency separately from energy intake, we pair-fed mice given a high-fat diet for 5 weeks. Body weight did not differ during pair feeding; however, fat mass was still increased, while fat-free mass was reduced in pair-fed MC3R hDM/hDM mice versus MC3R hWT/hWT ( Fig. 4c–e ). After switching from pair feeding to ad libitum diet, body weight significantly increased in MC3R hDM/hDM mice compared with MC3R hWT/hWT ( Fig. 4c ). These data indicate that alterations in both nutrient partitioning and energy intake contribute to the altered body composition and energy balance of MC3R hDM/hDM mice. 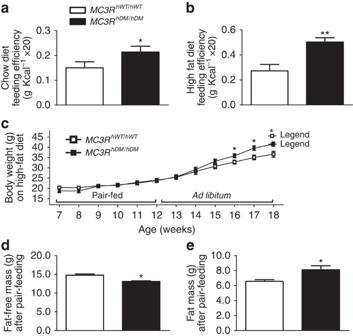Figure 4: Increased feeding efficiency inMC3RhDM/hDMmice. Feeding efficiency (the ratio of body weight to energy intake (g Kcal−1) × 20) was determined in femaleMC3RhWT/hWT(open bars) andMC3RhDM/hDM(closed bars) mice during (a) 5 weeks of chow diet feeding or (b) 7 weeks of high-fat-diet feeding. (c) For the high-fat pair-feeding study, the daily energy intake (11.83 Kcal per day) of 7- to 8-week-old female high-fat-fedMC3RhWT/hWTmice (n=7) was supplied to the age matched female high-fat-fedMC3RhDM/hDMmice (n=5), and their body weight change was monitored weekly. (d,e) Body composition ofMC3RhWT/hWTandMC3RhDM/hDMmice was determined immediately after the end of pair-feeding period at age 12–13 weeks. Data are represented as mean±s.e.m. *P<0.05 and **P<0.01MC3RhDM/hDMversusMC3RhWT/hWTmice. Groups were compared by Student'st-tests (two-tailed) (a,b,dande) and two-way analysis of variance followed by Bonferroni post-tests (c). Figure 4: Increased feeding efficiency in MC3R hDM/hDM mice. Feeding efficiency (the ratio of body weight to energy intake (g Kcal −1 ) × 20) was determined in female MC3R hWT/hWT (open bars) and MC3R hDM/hDM (closed bars) mice during ( a ) 5 weeks of chow diet feeding or ( b ) 7 weeks of high-fat-diet feeding. ( c ) For the high-fat pair-feeding study, the daily energy intake (11.83 Kcal per day) of 7- to 8-week-old female high-fat-fed MC3R hWT/hWT mice ( n =7) was supplied to the age matched female high-fat-fed MC3R hDM/hDM mice ( n =5), and their body weight change was monitored weekly. ( d , e ) Body composition of MC3R hWT/hWT and MC3R hDM/hDM mice was determined immediately after the end of pair-feeding period at age 12–13 weeks. Data are represented as mean±s.e.m. * P <0.05 and ** P <0.01 MC3R hDM/hDM versus MC3R hWT/hWT mice. Groups were compared by Student's t -tests (two-tailed) ( a , b , d and e ) and two-way analysis of variance followed by Bonferroni post-tests ( c ). Full size image To examine whether differences in energy expenditure contribute to the altered energy balance, we performed indirect calorimetry at 22 and 30 °C during chow and high-fat feeding using female MC3R hWT/hWT and MC3R hDM/hDM mice. During chow-feeding, total energy expenditure was significantly reduced in chow-fed MC3R hDM/hDM mice at thermoneutrality after adjusting for body weight ( Supplementary Table 2a ). However, total energy expenditure was not significantly different among chow-fed mice after adjusting for fat-free mass or fat-free mass and fat mass at 22 or 30 °C ( Supplementary Table 2a ). During high-fat feeding ( Supplementary Table 2b ), MC3R hDM/hDM mice, who exhibited no difference in total body weight compared with MC3R hWT/hWT , showed no significant change in total energy expenditure. Locomotor activity was also similar between groups during both chow and high-fat feeding ( Supplementary Table 2a,b ). Respiratory exchange ratio (RER) was significantly lower at 22 °C in chow-fed MC3R hDM/hDM mice ( Supplementary Table 2a ), but appeared to show a trend towards higher total RER ( P =0.07) at 30 °C in high-fat-fed MC3R hDM/hDM mice ( Supplementary Table 2b ), suggesting that altered substrate preference for generating energy does not appear to be a consistently applicable mechanism underlying the altered energy balance, since increased fat mass and reduced fat-free mass are found in both chow and high-fat-fed MC3R hDM/hDM mice. Leptin action Leptin resistance is observed in mice with high-fat-diet-induced obesity and many other mouse obesity models. Serum leptin concentrations increase in obese states and are accompanied by decreased responsiveness to exogenous leptin administration [20] . Because the MC3R is believed to be a downstream target of leptin signalling [21] , we examined leptin responsiveness using female MC3R hWT/hWT and MC3R hDM/hDM mice. We found increased serum leptin concentrations under both fasting and fed conditions in MC3R hDM/hDM mice ( Fig. 5a ). However, these differences were entirely accounted for by their increased fat mass ( Fig. 5b ). To examine whether decreased leptin responsiveness might explain the altered energy homeostasis of MC3R hDM/hDM mice, we injected body-weight-matched MC3R hDM/hDM and MC3R hWT/hWT mice (7–8 weeks old) with leptin. At this age, MC3R hDM/hDM mice already have greater fat mass than MC3R hWT/hWT mice ( Fig. 5e,f ). The leptin-induced decreases in body weight and energy intake were not significantly different between groups ( Fig. 5c,d ), indicating maintained leptin sensitivity in MC3R hDM/hDM despite their greater fat mass. These results suggest that inadequate leptin responsiveness does not explain why MC3R hDM/hDM mice exhibit alterations in energy intake behaviour. 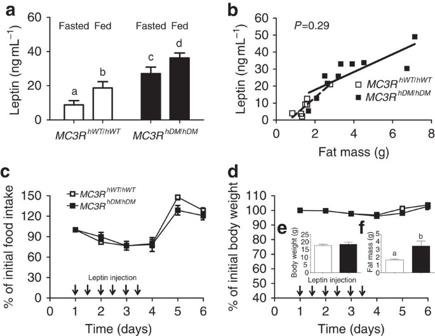Figure 5: Maintained leptin sensitivity inMC3RhDM/hDMmice. Blood was collected from tail veins of femaleMC3RhWT/hWT(open symbols) andMC3RhDM/hDM(closed symbols) mice. (a) Serum leptin concentrations were measured in fed (n=10 per group) and fasted (n=7 per group) conditions. (b) Serum leptin concentrations were significantly correlated with body fat mass in bothMC3RhWT/hWT(dotted line;P<0.0041) andMC3RhDM/hDM(solid line,P<0.0043) mice, but these slopes were not significantly different (P=0.29) and leptin values were not different after results were adjusted for fat mass. (c,d) 2-month-old chow-fed mice (n=5 per group) were injected twice daily with mouse leptin (1 μg g−1body weight, arrows) for 3 days. (c) Food intake and (d) body weight were measured daily. Inset bar graphs (e,f) show body weight and fat mass of the mice given leptin. Data are represented as mean±s.e.m. A different letter represents significant differences atP<0.05 compared with the other groups. Groups were compared by one-way (a) and two-way (c,d) analysis of variance followed by Bonferroni post-tests, Student'st-tests (two-tailed) (e–f), and analysis of covariance (b). Figure 5: Maintained leptin sensitivity in MC3R hDM/hDM mice. Blood was collected from tail veins of female MC3R hWT/hWT (open symbols) and MC3R hDM/hDM (closed symbols) mice. ( a ) Serum leptin concentrations were measured in fed ( n =10 per group) and fasted ( n =7 per group) conditions. ( b ) Serum leptin concentrations were significantly correlated with body fat mass in both MC3R hWT/hWT (dotted line; P <0.0041) and MC3R hDM/hDM (solid line, P <0.0043) mice, but these slopes were not significantly different ( P =0.29) and leptin values were not different after results were adjusted for fat mass. ( c , d ) 2-month-old chow-fed mice ( n =5 per group) were injected twice daily with mouse leptin (1 μg g −1 body weight, arrows) for 3 days. ( c ) Food intake and ( d ) body weight were measured daily. Inset bar graphs ( e , f ) show body weight and fat mass of the mice given leptin. Data are represented as mean±s.e.m. A different letter represents significant differences at P <0.05 compared with the other groups. Groups were compared by one-way ( a ) and two-way ( c , d ) analysis of variance followed by Bonferroni post-tests, Student's t -tests (two-tailed) ( e – f ), and analysis of covariance ( b ). Full size image Insulin sensitivity, serum lipid and hormone profiles Obesity is generally accompanied by a dysmetabolic syndrome that involves alterations in the hormones and substrates associated with insulin resistance [22] , [23] . We examined whether obese MC3R hDM/hDM mice have alterations in blood profile related to insulin sensitivity using female mice and found that serum triglycerides and cholesterol were, surprisingly, not significantly different in MC3R hWT/hWT versus significantly more adipose MC3R hDM/hDM mice examined under either chow-fed or fasted conditions ( Fig. 6a,b ). The serum concentrations of glucose and insulin were not significantly different between groups ( Fig. 6c,d ). Glucose and insulin-tolerance tests after high-fat diet feeding showed comparable responses for MC3R hDM/hDM mice versus MC3R hWT/hWT ( Fig. 6g,h ), suggesting that insulin sensitivity is relatively maintained in MC3R hDM/hDM mice despite their greatly increased adiposity ( Fig. 6i,j ). Similarly, no significant differences in serum triglycerides, free fatty acids (FFA) and insulin-tolerance test results were found in male MC3R hDM/hDM versus MC3R hWT/hWT mice (data not shown). 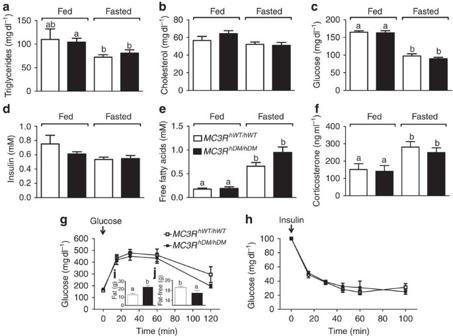Figure 6: Maintained insulin sensitivity and circulating lipid and hormone profile inMC3RhDM/hDMmice. Serum samples were used to measure (a) triglycerides, (b) total cholesterol, (c) glucose, (d) insulin, (e) free fatty acids and (f) corticosterone in 3-month-old femaleMC3RhWT/hWT(open symbols) andMC3RhDM/hDM(closed symbols) mice. ForMC3RhWT/hWTn=8 exceptn=6 for triglycerides and corticosterone; forMC3RhDM/hDMn=9. For glucose (g) and insulin (h) challenge tests (n=7 per group), glucose and insulin were injected at time 0. Fat mass (i) and fat-free mass (j) were determined on the day of the glucose tolerance test. Data are represented as mean±s.e.m. A different letter represents significant differences atP<0.05 compared to the other groups. Groups were compared with one-way (a–f) and two-way (g–h) analysis of variance followed by Bonferroni post-tests and Student'st-tests (two-tailed) (i,j). Figure 6: Maintained insulin sensitivity and circulating lipid and hormone profile in MC3R hDM/hDM mice. Serum samples were used to measure ( a ) triglycerides, ( b ) total cholesterol, ( c ) glucose, ( d ) insulin, ( e ) free fatty acids and ( f ) corticosterone in 3-month-old female MC3R hWT/hWT (open symbols) and MC3R hDM/hDM (closed symbols) mice. For MC3R hWT/hWT n =8 except n =6 for triglycerides and corticosterone; for MC3R hDM/hDM n =9. For glucose ( g ) and insulin ( h ) challenge tests ( n =7 per group), glucose and insulin were injected at time 0. Fat mass ( i ) and fat-free mass ( j ) were determined on the day of the glucose tolerance test. Data are represented as mean±s.e.m. A different letter represents significant differences at P <0.05 compared to the other groups. Groups were compared with one-way ( a – f ) and two-way ( g – h ) analysis of variance followed by Bonferroni post-tests and Student's t -tests (two-tailed) ( i , j ). Full size image It has been reported that a mechanism through which MC3R knockout mice increase fat mass and reduce lean mass is impaired fasting response, evidenced by lower fasting-induced adipose tissue lipolysis, higher basal corticosterone concentrations and diminished fasting-induced corticosterone [3] . However, basal FFA levels were not significantly different in the chow-fed condition, and fasting markedly increased serum FFA in both MC3R hWT/hWT and MC3R hDM/hDM mice ( Fig. 6e ). Similarly, fasting FFA concentrations were also not different between groups on a high-fat diet ( Supplementary Fig. 11a ). In addition, serum corticosterone was not different between groups in fasted and chow-fed conditions; fasting increased serum corticosterone in both MC3R hWT/hWT and MC3R hDM/hDM mice ( Fig. 6f ), indicating fasting-induced corticosterone response was maintained in MC3R hDM/hDM mice. Adiponectin Adiponectin is an adipocyte-derived hormone whose gene expression and blood concentrations are usually inversely associated with adiposity and insulin resistance [24] , [25] , [26] . Unexpectedly, both female and male MC3R hDM/hDM mice had significantly greater circulating adiponectin concentrations versus MC3R hWT/hWT under both fasted and chow-fed conditions ( Fig. 7a ; Supplementary Fig. 11c ) despite their notable increase in fat mass. On a high-fat diet, fat-mass-adjusted or non-adjusted fasting adiponectin was also significantly higher in female and male MC3R hDM/hDM mice, respectively ( Supplementary Fig. 11b,d ). These data indicate that MC3R sequence variants (C17A+G241A) paradoxically increase circulating adiponectin regardless of sex or nutritional state. 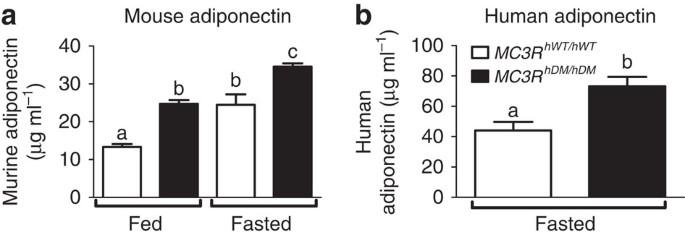Figure 7: Increased serum adiponectin inMC3RhDM/hDMmice and humans. (a) Serum adiponectin levels were measured in 3-month-old femaleMC3RhWT/hWT(open bars) andMC3RhDM/hDM(closed bars) mice under fed (n=8 per group) and fasted (n=11 per group). (b) Plasma samples from a matched cohort ofMC3RhWT/hWTandMC3RhDM/hDMchildren (Supplementary Table 4) were analysed for adiponectin (n=13 per group). Data are represented as mean±s.e.m. A different letter represents significant differences atP<0.05 compared with the other groups. Groups were compared by one-way analysis of variance followed by Bonferroni post-tests (a) and analysis of covariance (b). Figure 7: Increased serum adiponectin in MC3R hDM/hDM mice and humans. ( a ) Serum adiponectin levels were measured in 3-month-old female MC3R hWT/hWT (open bars) and MC3R hDM/hDM (closed bars) mice under fed ( n =8 per group) and fasted ( n =11 per group). ( b ) Plasma samples from a matched cohort of MC3R hWT/hWT and MC3R hDM/hDM children ( Supplementary Table 4 ) were analysed for adiponectin ( n =13 per group). Data are represented as mean±s.e.m. A different letter represents significant differences at P <0.05 compared with the other groups. Groups were compared by one-way analysis of variance followed by Bonferroni post-tests ( a ) and analysis of covariance ( b ). Full size image These findings led us to measure serum adiponectin in a cohort ( Supplementary Table 4 ) of age- and body-fat-matched children with homozygous wild type ( MC3R hWT/hWT , n =13) or homozygous double-mutant ( MC3R hDM/hDM , n =13) MC3R . Human subjects with MC3R hDM/hDM also had significantly greater serum adiponectin than those with MC3R hWT/hWT after adjusting for fat mass, sex and age ( P <0.01, Fig. 7b ). White adipose tissue adiponectin, PPARγ and phospho-AMPK Adiponectin is primarily secreted from white adipose tissues (WAT) [27] and WAT adiponectin expression is usually reduced in obesity [26] . To investigate the mechanism underlying the paradoxically increased adiponectin in MC3R hDM/hDM mice, we measured WAT adiponectin expression. WAT adiponectin mRNA ( Fig. 8a ) and protein ( Fig. 8c ) expression were not decreased in MC3R hDM/hDM mice despite their greater fat mass. Maintained adiponectin expression and secretion from the markedly increased adipose tissue mass of MC3R hDM/hDM mice may thus explain their increased circulating adiponectin. 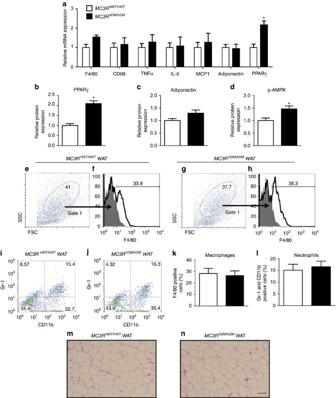Figure 8: Maintained adipose tissue function inMC3RhDM/hDMmice. Gonadal fat was isolated from fasted female mice fed a high-fat diet for (a) quantitative real-time PCR (MC3RhWT/hWTn=5;MC3RhDM/hDMn=8/group), (b–d) western blotting analysis (MC3RhWT/hWTn=5;MC3RhDM/hDMn=4), and (e–l) FACS analysis (MC3RhWT/hWTn=4;MC3RhDM/hDMn=5) inMC3RhWT/hWT(open bars) andMC3RhDM/hDM(closed bars) mice. (a) The expression levels of genes related to macrophage infiltration, inflammation and adipose tissue metabolism were normalized for β-actin expression. Western protein expression results for (b) peroxisome proliferator-activated receptor gamma (PPARγ), (c) adiponectin and (d) phosphospecific 5′-adenosine monophosphate-activated protein kinase (p-AMPK), divided by glyceraldehyde 3-phosphate dehydrogenase (GAPDH) expression and normalized relative to average forMC3RhWT/hWT. The stromal vascular fraction was isolated from gonadal fat (∼2 g) fromMC3RhWT/hWTandMC3RhDM/hDMmice. For detecting macrophages by flow cytometry, a gating strategy was used to enrich samples fromMC3RhWT/hWTandMC3RhDM/hDMmice for adipose tissue macrophages by selecting cells in the gate 1 area (e,g). The gate 1 area was stained with a F4/80 antibody (fandh) and the dot plots depict forward scatter (FSC) and side scatter (SSC) (left). For detecting neutrophils, whole cells (non-gated) were stained with CD11b and Gr-1 (i,j). Bar graphs show the average values±s.e.m. for percentage of cells in the stromal vascular fraction that were (k) macrophages and (l) neutrophils. *P<0.05MC3RhDM/hDMversusMC3RhWT/hWT. (m,n) Haematoxylin and eosin stained sections showed no apparent differences in adipocyte morphology between groups. Groups were compared by Student'st-tests (two-tailed) (a–dandk–i). Scale bar, 100 μm. Data are represented as mean±s.e.m. for a-d, k, and l. FACS, fluorescence-activated cell sorting Figure 8: Maintained adipose tissue function in MC3R hDM/hDM mice. Gonadal fat was isolated from fasted female mice fed a high-fat diet for ( a ) quantitative real-time PCR ( MC3R hWT/hWT n =5; MC3R hDM/hDM n =8/group), ( b – d ) western blotting analysis ( MC3R hWT/hWT n =5; MC3R hDM/hDM n =4), and ( e – l ) FACS analysis ( MC3R hWT/hWT n =4; MC3R hDM/hDM n =5) in MC3R hWT/hWT (open bars) and MC3R hDM/hDM (closed bars) mice. ( a ) The expression levels of genes related to macrophage infiltration, inflammation and adipose tissue metabolism were normalized for β-actin expression. Western protein expression results for ( b ) peroxisome proliferator-activated receptor gamma (PPARγ), ( c ) adiponectin and ( d ) phosphospecific 5′-adenosine monophosphate-activated protein kinase (p-AMPK), divided by glyceraldehyde 3-phosphate dehydrogenase (GAPDH) expression and normalized relative to average for MC3R hWT/hWT . The stromal vascular fraction was isolated from gonadal fat ( ∼ 2 g) from MC3R hWT/hWT and MC3R hDM/hDM mice. For detecting macrophages by flow cytometry, a gating strategy was used to enrich samples from MC3R hWT/hWT and MC3R hDM/hDM mice for adipose tissue macrophages by selecting cells in the gate 1 area ( e , g ). The gate 1 area was stained with a F4/80 antibody ( f and h ) and the dot plots depict forward scatter (FSC) and side scatter (SSC) (left). For detecting neutrophils, whole cells (non-gated) were stained with CD11b and Gr-1 ( i , j ). Bar graphs show the average values±s.e.m. for percentage of cells in the stromal vascular fraction that were ( k ) macrophages and ( l ) neutrophils. * P <0.05 MC3R hDM/hDM versus MC3R hWT/hWT . ( m , n ) Haematoxylin and eosin stained sections showed no apparent differences in adipocyte morphology between groups. Groups were compared by Student's t -tests (two-tailed) ( a – d and k – i ). Scale bar, 100 μm. Data are represented as mean±s.e.m. for a-d, k, and l. FACS, fluorescence-activated cell sorting Full size image The mRNA and protein levels of PPARγ, which is an essential factor for adipocyte differentiation, were significantly increased in WAT of MC3R hDM/hDM mice ( Fig. 8a,b ). Furthermore, the protein level of phosphorylated AMPK, which induces fatty acid oxidation, was significantly increased in WAT of MC3R hDM/hDM mice ( Fig. 8d ). White adipose tissue markers of inflammation Macrophages [28] , [29] and neutrophils [30] , [31] infiltrate into WAT in obesity, and this infiltration is associated with the development of insulin resistance. To examine WAT inflammation, we performed fluorescence-activated cell sorting on stromal vascular fractions isolated from WAT as well as WAT quantitative gene expression analysis. Measures of macrophage- (F4/80-positive cells) and neutrophil- (Gr-1 and CD11b double-positive cells) infiltration were not different in WAT of high-fat-fed MC3R hWT/hWT and MC3R hDM/hDM mice ( Fig. 8e–l ), despite the greater adiposity of MC3R hDM/hDM mice. In addition, the expression levels of macrophage markers (F4/80 and CD 68) and inflammatory genes (tumour necrosis factor α, interleukin-6 and MCP1) were not significantly changed in WAT of MC3R hDM/hDM versus MC3R hWT/hWT mice ( Fig. 8a ). H&E staining also showed no apparent differences in adipocyte morphology between groups ( Fig. 8m,n ). After collagenase digestion and isolation, however, adipocytes from the WAT of MC3R hDM/hDM had clearly increased lipid droplet size and cell diameter versus MC3R hWT/hWT (182±20 versus 132±20 μM, P =0.0002). Differentiation of mesenchymal stem cells MSCs are multipotent progenitor cells that can be differentiated to lineages of mesenchymal tissues including bone, fat and muscle [32] . Because MC3R hDM/hDM mice showed increased fat mass and decreased fat-free mass including a reduction in bone parameters including BMD and bone thickness, we hypothesized that MC3R hDM/hDM mice have altered MSC differentiation capacity, with a bias towards adipocytic lipid storing cells, instead of osteoblastic bone-forming cells. We therefore studied MSC differentiation capacity in MC3R hDM/hDM and MC3R hWT/hWT mice. To avoid potential contamination with haematopoietic stem cells, we isolated MSCs from compact bone including tibiae and femora of mice and confirmed the purity of MSCs by flow cytometry ( Supplementary Fig. 12 ). Western blotting showed that MC3R protein is expressed in MSCs ( Fig. 9a ). To investigate altered differentiation capacity, isolated MSCs were differentiated into osteoblasts or adipocytes and stained with Alizarin Red S (for calcium) and Oil Red O (for triglycerides). Differentiation into bone-forming osteoblasts was reduced ( Fig. 9b–f ) while differentiation into triglyceride-depositing adipocytes was significantly increased in MSCs of both male and female MC3R hDM/hDM mice compared with their wild-type counterparts ( Fig. 10a–c , data not shown for males). In addition, the mRNA expression of genes related to osteoblast differentiation such as BMP4, RUNX2 and collagen-α2 was significantly decreased ( Fig. 9k ) and the mRNA expression of genes related to adipocyte differentiation such as PPARγ, C/EBPα and FAS was markedly increased ( Fig. 10h ). Confocal imaging analysis further revealed that MSCs from MC3R hDM/hDM mice produced significantly less extracellular calcium deposits compared with their wild-type counterparts during osteoblast differentiation, although the levels of intracellular osteocalcin (osteoblast marker) were not significantly different among the groups ( Fig. 9g,j ). In contrast, during adipocyte differentiation, markedly increased lipid droplet formation was observed in MSCs obtained from the compact bone of MC3R hDM/hDM mice compared with MSCs from wild-type controls ( Fig. 10d–f ). Furthermore, the percentage of cells containing lipid droplets >10 μm in diameter was higher in cells derived from the MSCs of MC3R hDM/hDM during adipocyte differentiation ( Fig. 10g ). To further confirm the increased adipogenic capacity of MC3R hDM/hDM , we studied triglyceride accumulation in cells derived from the stromal vascular fraction (SVF) of adipose tissue, which is a rich source of preadipocytes, MSCs, endothelial progenitor cells and immune cells [33] . To minimize effects from other cell populations, we used an MSC differentiation medium believed to specifically differentiate adipogenic precursor cells into adipocytes. Cells from MC3R hDM/hDM SVF produced more lipid droplets after adipogenic stimulation compared to cells from MC3R hWT/hWT mice ( Supplementary Fig. 13a–e ). This result is consistent with the increase in PPARγ expression we found in MC3R hDM/hDM adipose tissue, since PPARγ is an essential factor for adipocyte differentiation from MSCs. These data further suggest there is increased adipogenic capacity in MC3R hDM/hDM compared with MC3R hWT/hWT mice. 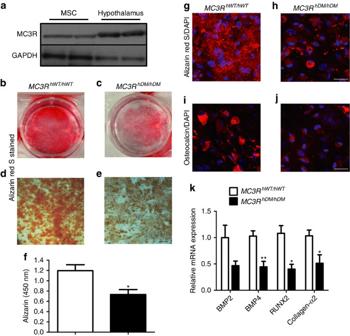Figure 9: Decreased osteoblast differentiation in MSCs ofMC3RhDM/hDMmice. MSCs were isolated from compact bone of tibia and femur from chow-fed femaleMC3RhWT/hWTandMC3RhDM/hDMmice at 7 weeks of age. Cells were isolated from one mouse for each group, and six independent experiments were performed (n=6/group). Isolated MSCs were cultured in 25-cm cell culture dishes for 4 passages (see methods for detailed information). MSCs were used (a) for western blotting to examine MC3R protein expression or (b–f) MSCs were differentiated into osteoblasts for 14 days to examine differentiation capacity. (b–c) Cultured MSCs differentiated into osteoblasts after Alizarin red S staining. (d–e) Microscopic images (10X) of osteoblasts after Alizarin red S staining. Scale bar, 100 μm. (f) Stained Alizarin red S was extracted from osteoblast and quantified at 450 nm. (g–j) Confocal microscopic images of osteoblasts stained with Alizarin red S (red) (g,h) or osteocalcin (red) (i,j). Nuclei were stained with DAPI (blue). Representative maximum intensity projection images are shown. Scale bar, 25 μm. (k) qPCR analysis of genes related to osteoblast differentiation (7 days after differentiation). Similar results were found for male mice (data not shown). Data are represented as mean±s.e.m. forfandk. Groups were compared by Student'st-tests (two-tailed) (f,k). Figure 9: Decreased osteoblast differentiation in MSCs of MC3R hDM/hDM mice. MSCs were isolated from compact bone of tibia and femur from chow-fed female MC3R hWT/hWT and MC3R hDM/hDM mice at 7 weeks of age. Cells were isolated from one mouse for each group, and six independent experiments were performed ( n =6/group). Isolated MSCs were cultured in 25-cm cell culture dishes for 4 passages (see methods for detailed information). MSCs were used ( a ) for western blotting to examine MC3R protein expression or ( b – f ) MSCs were differentiated into osteoblasts for 14 days to examine differentiation capacity. ( b – c ) Cultured MSCs differentiated into osteoblasts after Alizarin red S staining. ( d – e ) Microscopic images (10X) of osteoblasts after Alizarin red S staining. Scale bar, 100 μm. ( f ) Stained Alizarin red S was extracted from osteoblast and quantified at 450 nm. ( g – j ) Confocal microscopic images of osteoblasts stained with Alizarin red S (red) ( g , h ) or osteocalcin (red) ( i , j ). Nuclei were stained with DAPI (blue). Representative maximum intensity projection images are shown. Scale bar, 25 μm. ( k ) qPCR analysis of genes related to osteoblast differentiation (7 days after differentiation). Similar results were found for male mice (data not shown). Data are represented as mean±s.e.m. for f and k . Groups were compared by Student's t -tests (two-tailed) ( f , k ). 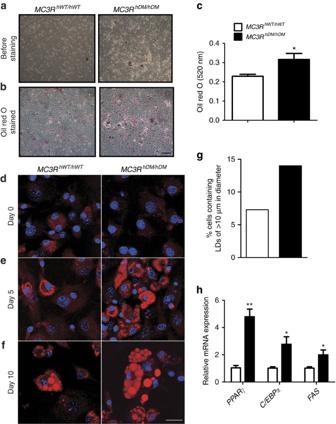Figure 10: Increased adipocyte differentiation in MSCs ofMC3RhDM/hDMmice. MSCs were isolated as described inFig. 8. (a–f) MSCs were differentiated into adipocytes to examine differentiation capacity. Cells were isolated from one mouse for each group, and six independent experiments were performed (n=6 per group). (a) Microscopic images (× 10) of MSCs differentiated into adipocytes for 18 days. (b) Microscopic images of differentiated adipocytes after Oil red O staining. Scale bar, 100 μm (c) Oil red O was extracted and quantified at 520 nm. (d–f) Confocal microscopic images of MSCs differentiated into adipocytes. Cells were stained with Nile Red and Hoechst 33342 at indicated days. Representative maximum intensity projection images of lipid droplets (LDs, red) and nuclei (blue) are shown. Scale bar, 25 μm (g) The percentage of cells displaying LDs>10 μm in diameter was quantified (n=∼350). (h) qPCR analysis of genes related to adipocyte differentiation (7 days after differentiation). Similar results were found for male mice (data not shown). Data are represented as mean±s.e.m. forcandh. Groups were compared by Student'st-tests (two-tailed) (c,h). Full size image Figure 10: Increased adipocyte differentiation in MSCs of MC3R hDM/hDM mice. MSCs were isolated as described in Fig. 8 . ( a – f ) MSCs were differentiated into adipocytes to examine differentiation capacity. Cells were isolated from one mouse for each group, and six independent experiments were performed ( n =6 per group). ( a ) Microscopic images (× 10) of MSCs differentiated into adipocytes for 18 days. ( b ) Microscopic images of differentiated adipocytes after Oil red O staining. Scale bar, 100 μm ( c ) Oil red O was extracted and quantified at 520 nm. ( d – f ) Confocal microscopic images of MSCs differentiated into adipocytes. Cells were stained with Nile Red and Hoechst 33342 at indicated days. Representative maximum intensity projection images of lipid droplets (LDs, red) and nuclei (blue) are shown. Scale bar, 25 μm ( g ) The percentage of cells displaying LDs>10 μm in diameter was quantified ( n = ∼ 350). ( h ) qPCR analysis of genes related to adipocyte differentiation (7 days after differentiation). Similar results were found for male mice (data not shown). Data are represented as mean±s.e.m. for c and h . Groups were compared by Student's t -tests (two-tailed) ( c , h ). Full size image To validate previous human studies that have suggested children with double-mutant (C17A+G241A) MC3R have greater fat mass [13] , [14] , [15] , we developed two humanized mouse models expressing human wild-type and double-mutant MC3R . We found that mice with MC3R hDM/hDM had altered nutrient partitioning, with increased body fat in adipose tissue and the bone marrow, along with decreased crown-rump length and reduced fat-free mass that was at least partially due to an alteration of MSC fate towards lipid accumulation instead of bone formation. Compared with the WAT of MC3R hWT/hWT , the WAT of MC3R hDM/hDM mice had increased protein expression of PPARγ and p-AMPK. Energy homeostasis was altered such that MC3R hDM/hDM mice demonstrated somewhat greater energy intake but also greater feeding efficiency, as is observed in Mc3r knockout mice. Finally, despite their greater adiposity, and unlike most obese mouse models, MC3R hDM/hDM mice had a reduction in expected obesity-associated metabolic dysfunction. MC3R hDM/hDM mice had greater circulating adiponectin, well-maintained insulin sensitivity, liver triglycerides and blood levels of metabolites and hormones that were similar to those of considerably less adipose MC3R hWT/hWT mice. In addition, the much larger WAT of MC3R hDM/hDM mice did not show greater immune cell infiltration or inflammation versus the WAT of MC3R hWT/hWT mice. These results suggest that the C17A+G241A human MC3R appears to stimulate an expansion of adipose tissue that is relatively metabolically healthy. Energy homeostasis is determined by the balance between energy intake and expenditure. Only total energy expenditure at thermoneutrality (30 °C) was significantly reduced in chow-fed MC3R hDM/hDM versus MC3R hWT/hWT mice after adjusting for body weight, but the differences between groups were not significant after adjusting for fat-free mass or when animals were studied in the high-fat-fed condition, indicating that the contribution of lower energy expenditure to the altered energy homeostasis, if any, may be subtle. This result is also similar to our prior human study [14] that found no differences in resting energy expenditure, total daily energy expenditure or RER among children with MC3R hWT/hWT and MC3R hDM/hDM . On the other hand, we found that energy intake was increased in MC3R hDM/hDM mice during both chow and high-fat feeding. Furthermore, we found no differences in body weight versus MC3R hWT/hWT mice during pair feeding, but an increase in body weight in MC3R hDM/hDM mice after switching from pair feeding to ad libitum intake, indicating that energy intake contributes to the altered energy balance. These data are also concordant with our previous human findings, that energy intake at a buffet meal was significantly higher in children with MC3R hDM/hDM compared with children who were heterozygous or homozygous for wild-type MC3R [14] . However, increased food intake is not the only mechanism underlying the altered energy metabolism in MC3R hDM/hDM mice because body composition was already changed during pair feeding before there were differences in total body weight. These data suggested changes in peripheral energy partitioning might contribute to the altered energy metabolism of MC3R hDM/hDM mice. In support of this hypothesis, it has been reported that increased feeding efficiency primarily contributes to the altered energy balance in MC3R knockout mice because energy intake is not consistently increased and energy expenditure is not altered in MC3R knockout mice [1] . In addition, when Mc3r is recovered only in the central nervous system of Mc3r knockout mice, such mice continue to demonstrate greater fat mass and less fat-free mass than controls [34] , indicating the potential importance of peripheral Mc3r signalling for altered nutrient partitioning. It is thus likely that changes in peripheral MC3R action contribute to the altered body composition of MC3R hDM/hDM mice. We hypothesized that altered Mc3r signalling could direct pluripotent MSC differentiation away from lean tissues and towards adipose tissue formation. Indeed, osteogenesis was notably reduced and lipogenesis was increased in MSCs of MC3R hDM/hDM mice. In addition, micro-CT analysis showed that femurs from MC3R hDM/hDM mice were shorter and had significantly reduced trabecular BMD and trabecular/cortical bone area in comparison to MC3R hWT/hWT mice. These data suggest that biasing MSC fate towards adipocytes instead of osteoblasts at least partially explains the increased fat mass and reduced bone mass of MC3R hDM/hDM mice. Multiple tissues may be used to isolate MSCs, including adipose tissue, bone and bone marrow. Our study showed that MSCs isolated from compact bone from MC3R hDM/hDM mice differentiated more readily into adipocytes rather than osteoblasts, but it is still unclear whether MSCs from bone contribute to the increase in adipose tissue mass in MC3R hDM/hDM mice. A human study indicates that bone marrow transplant can supply adipogenic progenitor cells to adipose tissue of the recipient [35] . Other studies indicate that MSCs can be mobilized and secreted into circulation [36] , [37] , [38] . These studies show the possibility that adipocyte precursor cells may be supplied through the circulation into adipose tissue. Furthermore, it has been reported that adiponectin stimulates MSC mobilization and secretion into circulation [39] . It is possible that increased adiponectin may stimulate MSC mobilization and provide new sources of adipocytes in adipose tissue of MC3R hDM/hDM mice. Adipocyte differentiation was also increased in cells derived from the SVF of MC3R hDM/hDM adipose tissue, showing the possibility that MSC characteristics in adipose tissue may also be changed in a manner similar to what we described for bone-derived MSCs. The specific alterations in MC3R function induced by MC3R hDM/hDM remain somewhat unclear. In vitro studies have suggested there is decreased MC3R protein expression and therefore partial inactivation of the MC3R after transient transfections of C17A+G241A MC3R [13] , [15] . However, other in vitro data suggest that C17A may actually reside in the 5′-UTR of the major MC3R transcript [17] , [18] . It is conceivable that C17A+G241A may change the balance of translation from the first and second in-frame ATGs and potentially interfere with MC3R function, for instance by altering its membrane localization [18] . Regardless, if the only change caused by MC3R hDM/hDM were decreased, but not absent, MC3R signalling, one might expect a phenotype similar to heterozygous MC3R knockout mice, which are not described as having marked changes in body composition. MC3R hDM/hDM does not appear to induce a functional knockout of MC3R; despite some phenotypic similarities, total Mc3r deficiency and MC3R hDM/hDM regulate tissue metabolism uniquely. For example, unlike Mc3r knockout mice, MC3R hDM/hDM mice, do not exhibit hyperglycaemia in low fat-fed conditions or increased inflammation in WAT in high-fat-fed conditions compared with wild-type mice [40] . Further studies are necessary to understand how the mutations studied may affect tissue-specific receptor expression, receptor stability, receptor trafficking and downstream signalling in both the central nervous system and peripheral tissues in vivo , but these results suggest a hitherto unrecognized role of MC3R signalling in adipocyte development. Obesity is generally associated with an impaired metabolic profile that includes changes in the hormones and substrates associated with insulin resistance [22] , [23] . However, MC3R hDM/hDM mice maintained serum lipid concentrations and insulin sensitivity comparable to those of MC3R hWT/hWT mice despite their increased fat mass and reduced fat-free mass. Our previous human study reported that the much more obese subjects we studied with MC3R hDM/hDM had serum glucose, triglycerides, total cholesterol and low-density lipoprotein cholesterol levels that were not significantly different from those of considerably less obese MC3R hWT/hWT children, although leptin and insulin were increased in proportion to fat mass among those with MC3R hDM/hDM [13] . The mechanisms through which obese MC3R hDM/hDM humans and mice avoid obesity-related metabolic dysfunction remain to be further established. The MSC-fate-driven expansion of metabolically healthy adipose tissue due to greater differentiation of stem cells into young adipocytes may contribute to this phenomenon, because it has been shown that the recruitment of adipogenic stem cells provides healthy adipose tissue expansion that is not involved in inflammation and systemic insulin resistance [41] . Adiponectin is an adipocyte-derived hormone that can improve insulin sensitivity and decrease inflammation [42] , [43] , whose gene expression and blood concentrations are normally inversely associated with body fat [25] . Surprisingly, despite the greater fat mass of MC3R hDM/hDM mice, we found increased serum adiponectin. We confirmed the same finding in a cohort of humans with MC3R hDM/hDM and MC3R hWT/hWT who were matched for demographic and anthropometric variables including body mass index and adiposity. It has been proposed that high adiponectin may serve as a ‘starvation’ signal in the hypothalamus that increases energy intake and reduces energy expenditure, thereby, counteracting leptin-mediated inhibition of energy intake [44] . Consistent with this view, a prior study has suggested that energy intake is a main regulator of circulating adiponectin [45] . The present study found that MC3R hDM/hDM mice maintained consistently higher adiponectin concentrations than MC3R hWT/hWT in both fasted and fed conditions. We also found that MC3R hDM/hDM mice exhibited higher leptin in circulation, but it was related to their enlarged adipose tissue rather than to the presence of primary leptin resistance. Thus, proximal leptin signalling pathway defects do not appear to contribute to the altered energy intake behaviour of MC3R hDM/hDM mice. It remains unclear why MC3R hDM/hDM mice have increased energy intake. One intriguing possibility is that the increased adiponectin of MC3R hDM/hDM mice may be mechanistically related to their greater food consumption and may play a role in maintaining their metabolic profile. Consistent with this hypothesis, when adiponectin is overexpressed in leptin-deficient mice, improvements in metabolic profile are accompanied by a remarkable expansion of adipose tissue [46] . Ob/ob mice that modestly overexpress adiponectin have increased PPARγ mRNA expression in WAT along with notable increases in WAT mass compared to ob/ob mice without adiponectin overexpression. The ob/ob mice with greater adiponectin also have ameliorated glucose and lipid profiles and reduced liver triglyceride and adipose tissue inflammation compared with ob/ob mice without adiponectin overexpression [46] . Similarly, we found that MC3R hDM/hDM mice showed increased PPARγ mRNA and protein expression in WAT, as well as WAT immune cell infiltration and inflammatory cytokine expression that were not exaggerated compared with that of less adipose MC3R hWT/hWT mice. The role of MC3R in regulating inflammation is not fully understood. However, some studies suggest that inhibiting MC3R signalling may potentially be beneficial to reduce inflammation. A clinical study found that during resistance training, which has been shown to reduce chronic inflammation, decreased MC3R expression in monocytes was significantly correlated with reduced C-reactive proteins levels, independent of changes in adiposity [47] . In addition, delayed macrophage infiltration is observed in WAT of high-fat-fed Mc3r knockout mice compared with Mc4r knockout mice [40] , [48] . Whether MC3R directly regulates immune cell function needs to be further elucidated. In conclusion, knock-in mice homozygous for human MC3R C17A+G241A have notably increased fat mass and reduced fat-free mass including decreased bone formation due to both greater energy intake and altered energy partitioning caused by MSC differentiation that is biased towards lipid-accumulating cells. These data help explain prior findings in humans of greater adiposity and energy intake among those homozygous for MC3R C17A+G241A. In mice, and at least in some respects among humans, the obese phenotype of MC3R hDM/hDM is associated with an amelioration of the metabolic dysfunction usually associated with obesity. Our study confirms the importance of MC3R signalling in human energy homeostasis and metabolism and suggests a unique mechanism underlying the early increase in fat mass observed in MC3R hDM/hDM mice and children with these MC3R mutations. Generation of human MC3R knock-in mice Mouse Mc3r was replaced by human wild-type or human double-mutant (C17A+G241A) MC3R ( Supplementary Fig. 1 ). The constructs for generating the two knock-in mouse lines were prepared by recombineering [49] . In brief, a targeting vector was constructed in the vector PKO Scrambler 916 (Stratagene, La Jolla CA). This vector contains a 5′ diphtheria toxin A negative selection cassette as well as a 3′ neomycin positive selection cassette that is flanked by loxP sites. At the ‘homology 1’ site (just 3′ to the negative selection cassette), we placed 2.978-kb genomic DNA (gDNA), comprising 1.895 kb of 5′ murine SV129 gDNA sequence upstream of the murine Mc3r start codon and 1.083 kb of the human MC3R sequence (either wild-type or C17A+G241A MC3R) . At the ‘homology 2’ site (3′ to the positive selection cassette), we placed 3.192 kb of 3′ murine SV129 genomic DNA sequence starting immediately after the mouse Mc3r stop codon. C57BL/6 ES cells were electroporated with the targeting vector and selected using G418. Positive clones were injected into C57BL/6 blastocysts to produce chimeras. Chimeric male mice were then mated with C57BL/6 female mice, and germline transmission was assessed by PCR. Mice with germline transmission of the knock-in alleles were then mated with C57BL/6- Gt (ROSA)26Sor tm16(Cre)Arte mice (Taconic, Hudson, NY) to delete the neomycin cassette, followed by further crossing with >10 generations of C57BL/6 nontransgenic ( MC3R +/+ ) mice, thereby creating heterozygous human MC3R double-mutant and wild-type mice in the C57BL/6 background. Heterozygous mice were crossed to obtain humanized homozygous, heterozygous and no construct mice. Genome scans (The Jackson laboratories, Bar Harbor, ME) with 155 single-nucleotide polymorphisms confirmed >99.5% identity with C57BL/6 for both knock-in mouse lines. All mice were maintained on a 12-h light, 12-h dark cycle and studied at 21–25 °C unless noted otherwise. Mice were fed either a chow diet (4.7% fat as calories, diet 7017, Harlan Laboratories, Frederick MD) or 45% high-fat diet (diet D12451, Research Diets, New Brunswick, NJ). All animal studies were conducted in accord with accepted standards of humane animal care under protocols approved by the NICHD or NIDDK Animal Care and Use Committees. There were no randomized or blinded experiments conducted. Identification of human plasma samples for adiponectin determination A cohort of 13 MC3R hDM/hDM and 13 MC3R hWT/hWT children was identified from among participants of prior clinical research studies ( http://www.clinicaltrials.gov/ct/show/NCT00001522 and http://www.clinicaltrials.gov/ct/show/NCT00001723 ) for whom a fasting plasma sample and body composition analysis by DXA were available for analysis. The human groups were selected to have similar age, race, sex, body mass index and adiposity ( Supplementary Table 4 ). All children gave written assent and parents gave written consent. The studies were approved by the Institutional Review Board of the Eunice Kennedy Shriver National Institute of Child Health and Human Development. Mouse body composition, indirect calorimetry and locomotor activity Body composition was determined using an EchoMRI mouse scanner (EchoMRI, Houston, TX) or using a PIXImus dual-energy X-ray absorptiometer (Lunar, Madison, WI), as indicated. Energy expenditure was measured at 22 and 30 ° C using a four-chamber Oxymax system (Columbus Instruments, Columbus, OH) as previously described, with one mouse per chamber [50] . On day 1 to day 2, mice were acclimated in the metabolic chamber at room temperature. On day 3, metabolic parameters were measured at 22 ° C for 24 h. On day 4, the temperature in the chamber was raised to 30 ° C in the morning, and measurements were begun 1 h later. Locomotor activity was determined at the same time that energy expenditure was measured using infrared beam interruption [50] . Micro-CT scanning To determine bone microarchitecture, the femurs from 12-week-old female MC3R hWT/hWT and MC3R hDM/hDM mice were isolated and scanned. Micro-CT was performed with the assistance of the NIH Mouse Imaging Facility using a Bruker MicroCT SkyScan 1172 Micro X-ray CT scanner (Micro Photonics, Inc. Allentown PA, USA, and Bruker MicroCT, Kontich, Belgium) with the X-ray source (focal spot size, 4 μm, energy range 20–100 kV) biased at 44 kV/267 μA and with a 0.5 mm Aluminium filter to reduce sample induced beam hardening. The images were acquired with a pixel size of 4.97 μm. Projections were acquired with an angular resolution of 0.5° through (180° or 360°) degrees rotation. Eight frames were averaged for each projection radiograph with an exposure time of 2,600 ms per frame. The scan duration was ∼ 2 h. Tomographic images were reconstructed filtered back projection using vendor-supplied software based on the Feldkamp cone beam algorithm. The data were calculated from the region of interest, which was defined as 0.503 mm offset from the growth plate; 2.753 mm height for trabecular bone, and 5.485 mm offset from growth plate; 0.418 mm height for cortical bone. The trabecular bone data include BMD, bone-volume fraction (BV/TV), trabecular number, trabecular thickness and trabecular separation. For cortical bone, data include total bone area (Tt.Ar), cortical area (Ct.Ar) and cortical area fraction (Ct.Ar/Tt.Ar) and mean cortical thickness. Immunoblots and quantitative real-time PCR For immunoblotting, mechanically homogenized tissue samples were separated using 4–12% NuPAGE gels (Invitrogen, Carlsbad, CA). Protein was blotted with antibodies for MC3R (SC 8990, Santa Cruz Biotechnology, Dallas, TX), PPARγ (SC 7273, Santa Cruz), GAPDH (SC 25778, Santa Cruz), p-AMPK (2535, Cell Signaling Technology, Danvers, MA) and adiponectin (MAB 1119, R&D Systems, Minneapolis, MN). Primary antibodies were diluted to 1:1000 concentration. Protein levels were semiquantified by image density scanning using Image J analysis (NIH, Bethesda, MD). The values were adjusted for GAPDH expression. For measuring MC3R protein expression, the hypothalamic N8 murine cell line, which does not express MC3R was used as a negative control [51] . Total RNA was prepared from gonadal fat and hypothalamus and homogenized with Trizol (Invitrogen, Carlsbad, CA). Genomic DNA was removed using RNAqueous kit (Ambion, Austin, TX) and complementary DNA was synthesized using SuperScript III first-strand (Invitrogen). Quantitative real-time PCR was performed using a 7900HT fast real-time PCR system (Applied Biosystems, Foster City, CA). For MC3R, BMP2, BMP4, RUNX2 and collagen-α2 gene expression, the Taqman gene expression system was used (HS 00252036 for Human MC3R , Mm 00434876 for mouse Mc3r , Mm 01340178 for BMP2 , Mm 00432087 for BMP4 , Mm 00501584 for RUNX2 and Mm 00483888 for collagen-α2 , Life Technologies, Grand Island, NY). For other gene expression studies, SYBR qPCR (4367659, Life Technologies, Grand Island, NY) was performed using the primers listed in Supplementary Table 3 . Flow cytometry Mouse gonadal fat pads ( ∼ 2 g) were minced and digested for 50 min at 37 °C with collagenase D (1 mg ml −1 ; Roche Applied Science, Indianapolis, IN) in DMEM containing 10% fetal bovine serum (pH 7.4) and 1% bovine serum albumin. After filtration of the digested fat through a nylon mesh (100 μM), the filtrate was centrifuged at 1,000 r.p.m. for 5 min. The SVF was obtained from the resulting pellet. SVF counts were determined with the Guava Viacount reagent in a Guava EasyCyte Mini System (Millipore, Billerica, MA). A gating strategy was used to enrich samples from MC3R hWT/hWT and MC3R hDM/hDM mice for adipose tissue macrophages by selecting cells in the gate 1 area (see Fig. 8e,g ) [52] . The proportion of macrophages was detected using mouse F4/80 antibody conjugated with fluorescein isothiocyanate (eBioscience, San Diego, CA) and the proportion of neutrophils was detected using mouse Gr-1 conjugated with fluorescein isothiocyanate, and mouse CD11b conjugated with phycoerythrin (eBioscience). Flow cytometry was conducted with a Guava EasyCyte Mini System (Millipore) using Guava CytoSoft Version 4.2.1 (Millipore) and FlowJo, Version 7 (TreeStar, Ashland, OR). Analysis of circulating metabolites and hormones Blood was collected from mouse tail veins cut with a scalpel blade in the fed or overnight-fasted (from 1800 hours to 0800 hours) condition and serum samples were prepared by centrifugation (4 °C) for 1,000–2,000 g for 10 min. Glucose was measured using a Glucometer Elite (Bayer, Elkhart, IN). Other metabolites or hormones were measured using the indicated kits; Insulin (SRI-13K, Linco Research, St Charles, MO), corticosterone (ADI-900-097; Enzo Life science, Farmingdale, NY), IGF-1 (22-IGF-R21, ALPCO, Salem, NH), Adiponectin (DRP 300 for human plasma samples obtained by venipuncture and MRP300 for mouse serum, R&D SYSTEMS, Minneapolis, MN), Leptin (MOB00, R&D SYSTEMS), triglycerides (337-B; Sigma), and non-esterified fatty acids (13831175; Roche Molecular Biochemicals, Indianapolis, IN). Triglyceride measurement Small pieces of liver were taken ( ∼ 0.3 g) for triglyceride measurement. For determination of bone marrow triglyceride content, both intact femurs were collected. The tips of the bones were cut to allow insertion of a 20-G needle at one end. Using a syringe, 20 ml of PBS was injected to flush bone marrow cells out of the marrow cavity and into a 50-ml conical tube. Cells were centrifuged at 1,200 r.p.m. for 5 min at room temperature. Eighten volumes of Hexane/2-propanol (3:2) solvent was added to each sample (liver and flushed bone marrow) followed by homogenization with tissue grinder. The lipid-containing layer was transferred to a new tube. After evaporation, the dried extract was reconstituted with 2-propanol. Triglycerides were measured using L-type TG M Microtiter Procedure (Wako Diagnostics, Richmond, VA, reagents 461-08992, 461-09092, 464-01601). Pair feeding, leptin treatment and glucose and insulin-tolerance tests A 5-week high-fat pair-feeding study was performed by supplying the daily energy intake (11.83 Kcal per day) of 7- to 8-week-old female high-fat-fed MC3R hWT/hWT mice to 7- to 8-week-old female high-fat-fed MC3R hDM/hDM mice. To study leptin sensitivity, mice were injected twice daily with mouse leptin (R&D Systems, Minneapolis, MN, 1 μg g −1 body weight, at 0730 hours and 1800 hours) for 3 days. To examine glucose homeostasis, glucose (2 g kg −1 ) or insulin (0.75 U kg −1 ) was injected intraperitoneally into fasted (from 1800 hours to 0800 hours for glucose) or fed (for insulin) female mice. Glucose was measured with a glucometer (Glucometer Elite, Bayer, Elkhart, IN). Mesenchymal stem cell isolation from mouse compact bone Mouse compact bones including tibiae and femurs were used to isolate MSCs rather than bone marrow tissues because hematopoietic cells still exist in bone-marrow-derived MSC cultures even after the preparation has been passaged nine times [53] . To obtain MSCs, 7- to 8-week-old mice were killed and soaked with 100 ml of 70% (vol/vol) ethanol for 5 min. Tibiae and femurs were isolated from both legs. The muscles and tendons were removed from tibiae and femurs using microdissecting scissors. Bone marrow was flushed out of the bones and the bones were minced with heavy-duty scissors (18054-11, Fine Science Tools, Foster City, CA) and digested with collagenase D (Roche Diagnostics, Indianapolis, IN). The digested bone fragments were cultured in 25-cm cell culture flasks with MSC basal media (Stem Cell Technologies, Vancouver, Canada) supplemented with MSC stimulatory supplement (Stem Cell Technologies, Vancouver, Canada) until it was passaged four times. Passaged MSCs underwent evaluation of purity by flow cytometry using CD29 (12-0291-83, ebioscience, San Diego, CA), CD106 (561613, ebioscience), CD44 (15-0441-83, ebioscience) and CD105 (12-1051-81, ebioscience) to detect pure MSCs and CD34 (primitive haematopoietic progenitor and endothelial cell marker) and CD45 (pan-leukocyte marker) for negative MSC markers (11-0341-85 and 15-0451-81, ebioscience) ( Supplementary Fig. 12 ). MSCs were differentiated into osteoblasts with osteogenic media (CCM 009, R&D system, Minneapolis, MN) for 14 days and into adipocytes with adipogenic media for 18 days (CCM 011, R&D system, Minneapolis, MN). Differentiated osteoblasts and adipocytes were stained with Alizarin Red S and Oil Red O respectively. Alizarin Red S and Oil Red O were then extracted from the cells using an osteogenesis quantitation kit (ECM 815, Millipore, Billerica, MA) and isopropanol respectively and quantified at 450 nm for Alizarin Red S and 520 nm for Oil Red O. Confocal microscopy Isolated MSCs (6 × 10 4 cells per well) were plated in Nunc Lab-Tek 1.5 Chambered 4 well Coverglass (Thermo Fisher Scientific Inc., Waltham, MA) and differentiated into adipocytes or osteoblasts as described earlier. At differentiation day 0, day 5 and day 10, cells were incubated with 0.00001% (vol/vol) Nile Red (Life Technologies, Grand Island, NY) and 1 μg ml −1 Hoechst 33342 (Life Technologies, Grand Island, NY) at 37 °C for 20 min to stain lipid droplets and nuclei, respectively. Afterwards, the cells were rapidly washed three times with prewarmed culture media. For osteoblast imaging, cells were fixed by using 4% paraformaldehyde in PBS at 37 °C for 15 min. After washing three times in PBS, cells were stained with Alizarin Red S as described earlier, or were blocked with PBS containing 3% bovine serum albumin and 0.3% TritonX100 (PBS-T) for 1 h at room temperature. Then, cells were incubated with 1/50 diluted osteocalcin antibody (SC 30045, Santa Cruz Biotechnology, Dallas, TX) in PBS-T at 4 °C for overnight. After washing three times in PBS for 5 min, the cells were treated with 1/500 diluted Alexa Fluor-conjugated secondary antibody (A 11060, Life Technologies) at 37 °C for 1 h. Then, the cells were incubated with 1 μg ml −1 DAPI (Life Technologies, Grand Island, NY) in PBS and were rinsed three times in PBS for 5 min. Images were acquired using Leica TCS SP5 (Leica Microsystems Inc., Buffalo Grove, IL). For imaging Nile Red and Hoechst 33342 (or DAPI), 561 nm white-light laser and 405-nm diode laser were used for excitation, and the emission signals were collected between 635–700 and 480–500 nm, respectively. For imaging Alizarin Red and endogenous osteocalcin, 546 nm white-light laser were used for excitation, and the emission signals were collected between 580 and 700 nm. ImageJ [54] was used to process and analyse images. Primary preadipocyte culture and adipocyte differentiation Epididymal adipose tissue was collected from 4- to 5-month-old female mice. Tissue was minced and incubated in DMEM with type I collagenase (30 mg per 4 g of tissue) at 37 °C for 1 h with gentle shaking. Samples were diluted 1:1 ratio into 10% FBS/DMEM after digestion, followed by filtration with 100 and 40 μM cell strainers to remove undigested tissues. Cells were centrifuged at 600 g for 7 min and the upper lipid layer and supernatant were discarded. Pellets were resuspended in 10 ml of 10% FBS/DMEM media, and 3–4 × 10 5 cells were plated into collagen pre-coated six-well plates. Media was changed on the next day and every 3 days until cells were differentiated into adipocytes. After 2 weeks, a special adipogenic medium (CCM 011, R&D system, Minneapolis, MN) was added for 2 weeks until Oil Red O staining. Statistical analysis Sample sizes were based on prior animal studies suggesting meaningful results from 5–15 animals per group. Data are expressed as mean±s.e.m. unless otherwise indicated. GraphPad Prism 5.0 software (GraphPad Software, San Diego, CA) was used for Student’s t -tests (two-tailed) and two-way analysis of variance followed by Bonferroni post-tests. IBM SPSS 18 software (Armonk, New York) was used for performing analysis of covariance for human adiponectin adjusted for age, sex and percentage fat mass and for adjusted energy intake and expenditure models for mice. Differences were considered significant at P <0.05. Data met assumptions of the statistical tests including requirements for similar variance across groups. Data are represented as mean±s.e.m. unless otherwise indicated. How to cite this article: Lee, B. et al . A mouse model for a partially inactive obesity-associated human MC3R variant. Nat. Commun . 7:10522 doi: 10.1038/ncomms10522 (2016).